Giant nonlinear optical activity in a plasmonic metamaterial In 1950, a quarter of a century after his first-ever nonlinear optical experiment when intensity-dependent absorption was observed in uranium-doped glass, Sergey Vavilov predicted that birefringence, dichroism and polarization rotatory power should be dependent on light intensity. It required the invention of the laser to observe the barely detectable effect of light intensity on the polarization rotatory power of the optically active lithium iodate crystal, the phenomenon now known as the nonlinear optical activity, a high-intensity counterpart of the fundamental optical effect of polarization rotation in chiral media. Here we report that a plasmonic metamaterial exhibits nonlinear optical activity 30 million times stronger than lithium iodate crystals, thus transforming this fundamental phenomenon of polarization nonlinear optics from an esoteric phenomenon into a major effect of nonlinear plasmonics with potential for practical applications. Since its discovery by François J.D. Arago in 1811 (ref. 1 ), optical activity, that is the ability to rotate the polarization state of light, has acquired great importance in spectroscopy, analytical chemistry, crystallography and molecular biology, and it is associated with the biochemistry of life [2] . It is now well understood that the effect is linked to chirality. In dissipative media optical activity manifests itself as circular birefringence, leading to polarization rotation, and circular dichroism, that is, differential transmission of circularly polarized waves, that yields a change of the degree of ellipticity of the propagating wave. In contrast to the Faraday effect, which causes polarization rotation in the presence of static magnetic fields, polarization rotation due to natural optical activity is reciprocal and it does not distinguish between opposite directions of wave propagation. The dependence of optical activity on the intensity of light was discussed by Vavilov in 1950 (ref. 3 ), a quarter of a century after the first effect of light self-action, the intensity-dependent absorption, was observed in uranium-doped glass [4] . The symmetry, wave propagation and quantum mechanical description of the phenomenon that later acquired the name of nonlinear optical activity (NOA) was then rigorously derived [5] , [6] , [7] , [8] , [9] , [10] , [11] . Observation of NOA due to the fast electronic mechanism of nonlinearity became possible in 1979, using a high-intensity single-mode nanosecond-pulsed laser and the natural crystal of lithium iodate that is simultaneously a highly nonlinear and strongly optically active medium [12] ( Fig. 1a ). Shortly after that, transient pump-probe measurements of NOA were performed in the chiral cholesteric phase of a liquid crystal exploiting the thermal mechanism of nonlinearity [13] . Thermal NOA was also seen in optically active crystals [14] , [15] , [16] . Since then NOA has been observed in a number of chiral liquids [17] , [18] , [19] , [20] . Nevertheless, the effect remained challenging to detect, making it unsuitable for routine practical applications, even in spectroscopy. 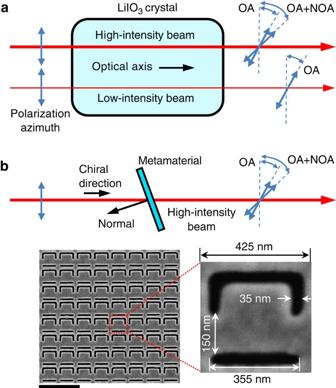Figure 1: Nonlinear optical activity. (a) To observe NOA in 1979 in a LiIO3crystal, intensity-dependent change of the polarization azimuth of about 0.02° was recovered on a background of 8,000° of natural rotation by comparing the polarization state in high-and-low intensity channels using a pulsed laser12. (b) Observation of NOA in a gold plasmonic metamaterial along a chiral direction, where nonlinearity is resonantly enhanced by nanoscale confinement of light. The scanning electron micrograph shows a fragment of the gold nanostructure (1-μm scale bar) and detailed dimensions of a single meta-molecule. Figure 1: Nonlinear optical activity. ( a ) To observe NOA in 1979 in a LiIO 3 crystal, intensity-dependent change of the polarization azimuth of about 0.02° was recovered on a background of 8,000° of natural rotation by comparing the polarization state in high-and-low intensity channels using a pulsed laser [12] . ( b ) Observation of NOA in a gold plasmonic metamaterial along a chiral direction, where nonlinearity is resonantly enhanced by nanoscale confinement of light. The scanning electron micrograph shows a fragment of the gold nanostructure (1-μm scale bar) and detailed dimensions of a single meta-molecule. Full size image Although NOA in natural media was weak, hopes have been growing that a stronger effect could be found in artificial media. Indeed, an observation of optical activity in artificial media (twisted jute) in the millimeter wave part of the spectrum was reported by J.Bose as far back as 1898 (ref. 21 ). Recently, with the development of metamaterials (periodic media structured on the subwavelength scale), it has become possible to design optimized photonic structures with specific optical activity orders of magnitude larger than in natural media [22] , [23] , [24] , [25] . It was found, for instance, that artificial circular birefringence could be so strong that, whereas it is normally a correction to the refractive index, in some metamaterials it makes the refractive index negative for one circular polarization [26] , [27] . Moreover, recent experiments in waveguides revealed that a chiral inclusion containing a varactor nonlinear element forces a strong intensity-dependent rotation of the polarization state of microwave radiation and exhibits asymmetric transmission [28] . At the same time, resonant local field enhancement in plasmonic metamaterials can dramatically amplify the nonlinear response of hybridized materials, such as silicon [29] , [30] and carbon nanotubes [31] , and even the metal forming the metamaterial framework itself [32] , [33] . The phenomenon of natural optical activity is inextricably linked to chirality. In many optically active media, chirality resides in the left–right asymmetry of the constituent components of the medium. For instance, a liquid consisting of only one form of chiral molecules, that is, molecules that are not congruent with their mirror image, is likely to exhibit optical activity. Here the best known natural example is sugar solution where optical activity is routinely used to measure the concentration of the syrup. Optical activity may also result from chiral arrangements of non-chiral molecules, as it may be found in crystals of quartz or lithium iodate. Chirality can also emerge from the mutual arrangement of the beam of light and the medium, creating what is known in crystallography as a screw direction. For instance a regular array of oriented molecules that are not chiral in their own right, could make an arrangement with a beam of light that lacks mirror symmetry and shows optical activity [34] , [35] . In general, only crystals whose point group contains no inversion centre could have screw directions. Polarization rotation in certain symmetric crystal classes is underpinned by this mechanism of optical activity [36] , which is also routinely observed in liquid crystals [37] and metamaterials [38] . True circular birefringence and dichroism can be found in these cases. Here we report that a plasmonic metamaterial exhibits a huge NOA in the optical part of the spectrum. It is 30 million times stronger than in the lithium iodate crystal [12] . This colossal magnitude of the nonlinear polarization effect was achieved by combining strong metamaterial optical activity due to extrinsic chirality with strong metamaterial optical nonlinearity: in this artificial medium, the figure of merit that represents specific nonlinear polarization rotation (° per cm) per unit of optical intensity (W cm −2 ) is 3×10 −4 °cm W −1 (compare with 10 −11 °cm W −1 for lithium iodate). As a result, nonlinear rotation on the order of degrees can be seen at an average laser power level of only a few milliwatts. Optical activity due to extrinsic chirality The metamaterial consists of a periodic array of asymmetric split ring slits, which were cut by focussed ion-beam milling through a 50 nm thick gold film supported by a 500 μm thick fused quartz substrate. The overall size of the metamaterial array is 100 ×100 μm 2 with a period of 425 nm, and the individual meta-molecules lack inversion symmetry ( Fig. 1b ). 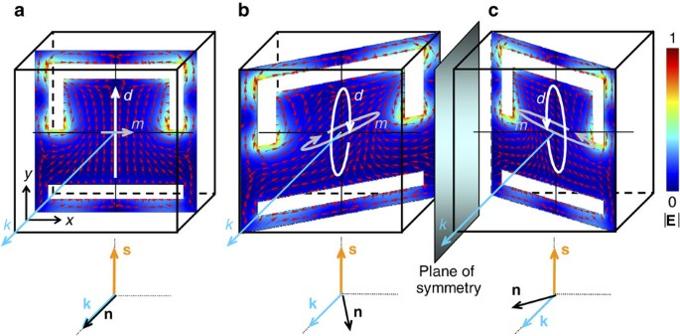Figure 2: Chiral scattering in plasmonic metamaterial. Electric field magnitude |E| (colour map) and instantaneous directions of the electric field (small red arrows) inside the metamaterial gold film, for excitation withy-polarized light at (a) normal incidence, (b) +20° oblique incidence (experimental case) and (c) −20° oblique incidence. At normal incidence, the unit cell's total electricdand magneticmdipoles trace perpendicular directions. No polarization change is observed in this case (a). At oblique incidence, vectorsdandmtrace ellipses with main axes that are not perpendicular to one another. The scattered wave's polarization is now different from that of the incident wave. The polarization change reverses with reversing sense of chirality of the mutual arrangement of the incident light wave (vectork) and the metamaterial's normalnand symmetry axiss; scenarios (b) and (c) are mirror-symmetric and will show optical activity equal in amplitude but opposite in sign. Figure 2 illustrates the origin of chirality and optical activity in this material for oblique incident angles. It is caused by circular differential forward scattering of incident photons that may be traced down to the scattering contributions of the unit cell's effective electric d and magnetic m dipole moments induced by the incident wave. It is well known from the molecular theory that optical activity requires the molecule to exhibit magnetic and electric responses simultaneously in such a way that there is a non-zero projection of the induced magnetic dipole on the induced electric dipole [2] , [39] . In this case, the forward scattered wave will exhibit polarization rotation, as electric and magnetic dipoles will emit orthogonal polarization components with a phase lag. The mechanism for extrinsic chirality in metamaterials is illustrated by the finite element method simulations in Fig. 2 for a single meta-molecule excited by an incident y -polarized wave. At normal incidence, the field distribution in the unit cell of the metamaterial is mirror-symmetric with respect to the y -direction. The total electric and magnetic moments of the unit cell oscillate along strictly perpendicular directions; no optical activity is observed in this case ( Fig. 2a ). At oblique incidence, the total induced magnetic and electric moments are tracing ellipses, whose main axes are no longer perpendicular and conditions are right for the meta-molecule to scatter with a polarization change. This polarization effect is optical activity and it will change sign with changing chirality of the arrangement, as illustrated by Fig. 2b,c . Figure 2: Chiral scattering in plasmonic metamaterial. Electric field magnitude | E | (colour map) and instantaneous directions of the electric field (small red arrows) inside the metamaterial gold film, for excitation with y -polarized light at ( a ) normal incidence, ( b ) +20° oblique incidence (experimental case) and ( c ) −20° oblique incidence. At normal incidence, the unit cell's total electric d and magnetic m dipoles trace perpendicular directions. No polarization change is observed in this case ( a ). At oblique incidence, vectors d and m trace ellipses with main axes that are not perpendicular to one another. The scattered wave's polarization is now different from that of the incident wave. The polarization change reverses with reversing sense of chirality of the mutual arrangement of the incident light wave (vector k ) and the metamaterial's normal n and symmetry axis s ; scenarios ( b ) and ( c ) are mirror-symmetric and will show optical activity equal in amplitude but opposite in sign. Full size image Measurements of linear optical activity and anisotropy We studied linear and intensity-dependent optical activity using a femtosecond mode-locked tunable laser with 115 fs pulse duration and 80 MHz repetition rate. 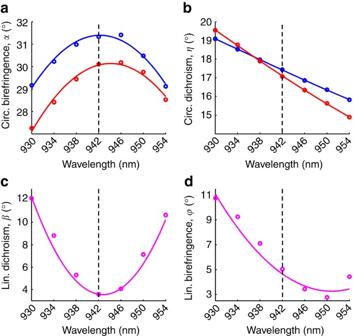Figure 3: Giant linear polarization effects in a plasmonic nanostructure. Optical activity in terms of (a) circular birefringence (polarization rotation) and (b) circular dichroism (ellipticity angle) at linear and nonlinear average power levels of 50 μW (blue) and 5 mW (red), respectively; optical anisotropy in terms of (c) linear dichroism and (d) linear birefringence at 50 μW average power. Vertical dashed lines indicate the wavelength of 942 nm for which the power dependence of NOA has been studied. Figure 3 illustrates the metamaterial's linear (low-power) optical properties for wavelengths between 930 and 954 nm, where the metamaterial has a plasmonic resonance and optical activity is largest. In general, in media of low symmetry optical activity coexists with anisotropy that manifests itself as differential refraction (birefringence) and transmission (dichroism) for orthogonal linear polarizations. Figure 3: Giant linear polarization effects in a plasmonic nanostructure. Optical activity in terms of ( a ) circular birefringence (polarization rotation) and ( b ) circular dichroism (ellipticity angle) at linear and nonlinear average power levels of 50 μW (blue) and 5 mW (red), respectively; optical anisotropy in terms of ( c ) linear dichroism and ( d ) linear birefringence at 50 μW average power. Vertical dashed lines indicate the wavelength of 942 nm for which the power dependence of NOA has been studied. Full size image On propagation through an optically active and anisotropic medium, a wave with initially linear polarization becomes elliptically polarized and its polarization azimuth rotates. For moderate polarization changes, it may be shown that rotation of the polarization azimuth contains contributions resulting from circular birefringence α and linear dichroism β , while the ellipticity of the transmitted wave will contain contributions from circular dichroism η and linear birefringence φ . These four contributions can be separated by measuring polarization rotation and ellipticity angle as functions of the input polarization azimuth of an initially linearly polarized wave, providing α , β , η , φ ≪ π (see Methods). Figure 3 presents measurements of circular birefringence and dichroism (optical activity) and linear birefringence and dichroism (anisotropy) in the metamaterial sample, observed as functions of wavelength at the incident angle of 20° to the normal (measurements taken at −20° show rotation and ellipticity angles of the same magnitude but opposite signs). We note that optical activity is the dominant contribution to the polarization azimuth and ellipticity changes at the resonance wavelength of 942 nm; here anisotropy contributes only up to 12% to the total polarization azimuth rotation and 30% to ellipticity. Detailed measurements of the intensity-dependent polarization changes, reported below, were performed at this wavelength. Measurements of nonlinear optical activity The intensity dependence of optical activity was studied using the same laser source as for the linear characterization. While we performed the linear measurements at an average power of 50 μW, the laser power was ramped up to 5 mW for nonlinear measurements, which corresponds to a peak intensity of I =2 GW cm −2 as the beam is focused to a spot size of 8 μm in diameter. This is sufficient to see a profound change of the light polarization state with intensity, as illustrated by Fig. 4a,b . Here results are represented in terms of changes relative to the low-intensity values of circular birefringence Δ α and circular dichroism Δ η . The most obvious effect of increasing intensity is a suppression of optical activity; at 942 nm polarization rotation is reduced by 1.0°, whereas the ellipticity angle drops 0.5°. 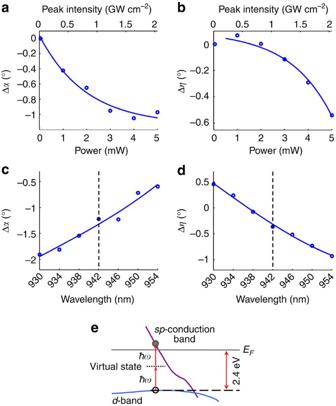Figure 4: Nonlinear optical activity of a plasmonic metamaterial. Power-dependent changes of the metamaterial's (a) circular birefringence Δαand (b) circular dichroism Δηfor a fixed wavelength of 942 nm. Spectral dependence of nonlinear (c) circular birefringence and (d) circular dichroism for a fixed average power of 5 mW (relative to 50 μW in all cases; guides to the eye are shown alongside experimental data points). The wavelength of 942 nm, for which the power dependence of NOA has been studied, is marked by dashed lines. (e) Sketch of the Au-band structure and the two-photon absorption process, where ad-band electron is excited to thesp-conduction band above the Fermi levelEFvia absorption of two photonsω. Figure 4: Nonlinear optical activity of a plasmonic metamaterial. Power-dependent changes of the metamaterial's ( a ) circular birefringence Δ α and ( b ) circular dichroism Δ η for a fixed wavelength of 942 nm. Spectral dependence of nonlinear ( c ) circular birefringence and ( d ) circular dichroism for a fixed average power of 5 mW (relative to 50 μW in all cases; guides to the eye are shown alongside experimental data points). The wavelength of 942 nm, for which the power dependence of NOA has been studied, is marked by dashed lines. ( e ) Sketch of the Au-band structure and the two-photon absorption process, where a d -band electron is excited to the sp -conduction band above the Fermi level E F via absorption of two photons ω . Full size image To determine the strength of NOA, we shall be concerned with the gradient of the polarization azimuth rotation change with increasing incident intensity that is measured to be about Δα/I=−0.8°cm 2 per GW, before nonlinear rotation starts to saturate above 1 GW cm −2 . Here nonlinearity resides in the gold film of thickness 53 nm along the direction of propagation. Thus, the specific constant of NOA is Ω =3×10 −4 °cm W −1 (this accounts for the 50% reflection of the metamaterial sample). This is more than 7 orders of magnitude stronger than NOA in natural materials such as LiIO 3 (10 −11 °cm W −1 (ref. 12 )), sucrose (2×10 −11 °cm W −1 (refs 17 , 20 )), α -pinene (≤10 −11 °cm W −1 (ref. 20 )) and ruthenium salt solution [18] , [19] . The spectral dependence of NOA is shown by Fig. 4c,d . Nonlinear circular birefringence becomes more pronounced towards shorter wavelengths, whereas nonlinear circular dichroism changes sign at about 937 nm. As illustrated by Fig. 3a , the increase of light intensity reduces the overall polarization rotation throughout the studied spectral range. The nonlinearity of the metamaterial resides in the nonlinearity of its metal framework. It is mainly caused by the nonlinear process of direct two-photon absorption between the d and sp states in the gold band structure ( Fig. 4e ). Here direct two-photon absorption occurs through a virtual state when the energy ω of two incident photons is combined to bridge the gap Δ E =2.4 eV, between the d states and states above the Fermi level: Δ E /2< ω <Δ E . As the energy gap cannot be bridged by individual photons directly, 'Fermi-smearing', which dominates the nonlinearity of gold in the visible, is less important in our case. This inherited nonlinearity of gold is resonantly enhanced more than 300 times by the nanostructure through the virtue of strong field concentration at the edges of the grooves, which support a plasmonic mode (see bright hot-spots of field maps in Fig. 2 ) [32] . Pump-probe experiments [32] also confirmed that this is a very fast nonlinearity, because its main mechanism requires both the pump and the probe photons to be present simultaneously. This degenerate cubic optical nonlinearity gives rise to a nonlinear absorption coefficient on the order of 10 −5 m W −1 . Importantly, the spectral maxima of the absorption nonlinearity and optical activity in this metamaterial overlap, as they are underpinned by the same plasmonic resonance, which arises from the asymmetry of the metamaterial pattern [25] , [32] . The asymmetry of the plasmonic structure results in excitation of a strong anti-phased current mode through weak free-space coupling, which ensures low radiation losses and therefore a narrow Fano-type optical resonance [40] . Here two-photon absorption reduces not only the intensity of light transmitted through the nanostructure, but it also hampers the chiral dipole scattering efficiency by dampening the underlying plasmon oscillations. Manifestation of this is a suppression of circular birefringence at high intensities ( Fig. 3a ). It may be expected that similarly large nonlinear polarization effects can be observed at resonances in a wide range of plasmonic metamaterials. In particular, large NOA may also occur in intrinsically three-dimensionally chiral metamaterials while chiral plasmonic interfaces [41] may show nonlinear versions of other polarization effects such as asymmetric transmission [42] . In summary, we report that engineering of chiral and nonlinear optical properties in a plasmonic metamaterial allows the observation of NOA that is millions of times stronger than in natural crystals. Observation of this giant polarization effect provides a powerful illustration that nanoscale nonlinear plasmonics of metamaterials offers extremely strong effects unfolding in nanoscale volumes of nonlinear medium that could lead to applications in modulation of light intensity and polarization in nanophotonic devices. Definition of polarization parameters The polarization state of polarized light is characterized by the polarization azimuth Φ and the ellipticity angle ζ which are defined by the polarization ellipse, that is, the trace of the end of the electric field vector as seen by an observer looking into the beam ( Fig. 5a ). 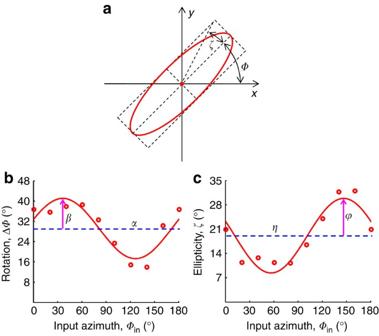Figure 5: Measuring optical activity and optical anisotropy. (a) Polarization azimuthΦand ellipticity angleζof the polarization ellipse (red) define the polarization state of a polarized electromagnetic wave. (b) Polarization azimuth rotation ΔΦ and (c) ellipticity angleζas a function of the azimuthΦinof the linearly polarized incident wave. The individual contributions of circular birefringenceαand circular dichroismηcorrespond to the average levels of rotation and ellipticity of the transmitted wave, while the corresponding modulations arise from linear dichroismβand linear birefringenceφ, respectively. The data shown was taken at 20° oblique incidence for a wavelength of 930 nm and low average power (50 μW). Figure 5: Measuring optical activity and optical anisotropy. ( a ) Polarization azimuth Φ and ellipticity angle ζ of the polarization ellipse (red) define the polarization state of a polarized electromagnetic wave. ( b ) Polarization azimuth rotation ΔΦ and ( c ) ellipticity angle ζ as a function of the azimuth Φ in of the linearly polarized incident wave. The individual contributions of circular birefringence α and circular dichroism η correspond to the average levels of rotation and ellipticity of the transmitted wave, while the corresponding modulations arise from linear dichroism β and linear birefringence φ , respectively. The data shown was taken at 20° oblique incidence for a wavelength of 930 nm and low average power (50 μW). Full size image Separation of optical activity and optical anisotropy On propagation through an optically active and anisotropic medium, a wave with initially linear polarization becomes elliptically polarized and its polarization azimuth rotates. For moderate polarization changes, it may be shown that the polarization azimuth change Δ Φ contains contributions resulting from circular birefringence α and linear dichroism β . On the other hand, the ellipticity angle ζ of the initially linearly polarized wave after interacting with the sample will contain contributions from circular dichroism η and linear birefringence φ . Indeed, in the slow envelope approximation, evolution of the polarization state of light in linear media is governed by the following set of equations for the components of the four-dimensional Stokes vector S , which in a Cartesian coordinate frame can be written as follows (formula 3.24, ref. 10 ): Here z is the propagation direction, k and ω are the wave number and frequency, c is the speed of light, E is the electric field vector, σ α are Pauli spin matrices, δ ij is the Kronecker delta, and (formulae 3.19 and 3.21, ref. 10 ) where are cartesian components of the dielectric coefficient describing anisotropy and Γ ijz are cartesian components of the nonlocality tensor describing optical activity. They are defined by the constitutive equation for the nonlocal anisotropic response (formula 2.14, ref. 10 ): Therefore, it follows from the linear nature of equation (1) that small changes of the Stokes vector components and, thus, small polarization changes that are induced by the anisotropic and nonlocal effects are additive. Now, by measuring the sample's polarization rotation Δ Φ and ellipticity angle ζ as functions of the input polarization azimuth Φ in of an initially linearly polarized wave, one can separate these four contributions, providing α , β , η , ≪ π . Precise formulae for these contributions are given by formulae 3.41, 3.48 and 3.49 in ref. 10 . For our consideration, here it is important that, for initially linearly polarized waves, polarization rotation and induced ellipticity are proportional to Re( Γ xyz ) and Im( Γ xyz ) describing circular birefringence and circular dichroism, correspondingly. Polarization rotation and induced ellipticity also have components that oscillate with the incident polarization azimuth Φ in as sin(2 Φ in ). They are proportional to linear dichroism described by Im( − ) and linear birefringence described by Re( − ). Within this approximation, we retrieve circular birefringence α by measuring the Φ in -independent (average) component of the polarization azimuth rotation; we retrieve circular dichroism η by measuring the Φ in -independent (average) component of the ellipticity angle; we retrieve data on linear birefringence φ by measuring the amplitude of oscillation of the ellipticity angle with the incident polarization azimuth; we retrieve data on linear dichroism β by measuring the amplitude of oscillation of the polarization azimuth rotation with the incident polarization azimuth ( Fig. 5b,c ). How to cite this article: Ren, M. et al . Giant nonlinear optical activity in a plasmonic metamaterial. Nat. Commun. 3:833 doi: 10.1038/ncomms1805 (2012).